Mitochondrial inner membrane protease promotes assembly of presequence translocase by removing a carboxy-terminal targeting sequence The presequence translocase of the inner mitochondrial membrane (TIM23 complex) is essential for importing cleavable preproteins into mitochondria. The preproteins contain amino-terminal targeting sequences that are removed by the mitochondrial processing peptidase (MPP). Some preproteins carry bipartite presequences that are cleaved twice, by MPP and the inner membrane protease (IMP). Here, we report that the TIM23 complex is altered in mitochondria lacking the IMP subunit Imp1 although none of the TIM23 components contains a bipartite presequence. We show that the TIM23 subunit Mgr2 is processed by IMP, but not by MPP. The cytosolic precursor of Mgr2 contains a carboxy-terminal sequence that promotes targeting to mitochondria, but impairs stable assembly and function of the mature TIM23 complex. IMP removes the carboxy-terminal targeting sequence and thus promotes proper assembly of the TIM23 complex. Our results reveal carboxy-terminal processing as a new mechanism in the biogenesis of the mitochondrial inner membrane. The vast majority of mitochondrial proteins are synthesized as precursors on cytosolic ribosomes. The precursor proteins contain targeting signals that direct them to mitochondria. Protein translocation machineries import the precursor proteins and sort them to their functional sites in the organelle [1] , [2] , [3] , [4] , [5] , [6] , [7] , [8] . Depending on their intramitochondrial location, precursor proteins carry different types of targeting sequences, either as cleavable amino-terminal extensions or as non-cleavable signals that are embedded in the mature part of the proteins [3] , [4] , [7] , [8] . Presequences represent the most frequent type of mitochondrial-targeting signals [9] , [10] , [11] . They form positively charged amphipathic α-helices at the N termini of preproteins and direct them to the mitochondrial matrix. Presequences are also used by proteins destined for the inner membrane or intermembrane space when the proteins include a hydrophobic sorting sequence that arrests translocation in the inner membrane [3] , [4] , [12] , [13] . Presequence-carrying proteins are imported by the general translocase of the outer mitochondrial membrane (TOM complex) and are handed over to the presequence translocase of the inner membrane (TIM23 complex). The TIM23 complex consists of three core components, the inner membrane proteins Tim17, Tim23 and Tim50 (refs 3 , 4 , 6 ). Two further subunits of the TIM23 complex, Tim21 and Mgr2, are involved in coupling the TIM23 complex to the TOM complex as well as to the respiratory chain [14] , [15] , [16] , [17] , [18] . Two main species of the TIM23 complex can be distinguished, a TIM23 CORE complex that consists of Tim17, Tim23 and Tim50 and a larger TIM23 SORT complex that additionally includes Tim21 and Mgr2 (refs 14 , 17 , 19 , 20 ). The TIM23 SORT complex is sufficient for the membrane potential-driven lateral insertion of preproteins into the inner membrane [20] , whereas the complete translocation of preproteins into the matrix requires cooperation of the TIM23 machinery with the presequence translocase-associated motor (PAM) [3] , [14] , [16] , [18] , [19] , [21] , [22] . Nearly all presequences are proteolytically processed by the matrix-located presequence-specific mitochondrial processing peptidase (MPP) [3] , [10] , [23] , [24] . For a number of preproteins, a second processing event takes place. Several specific proteases have been identified that act on preprotein intermediates generated by MPP [11] , [24] . The matrix intermediate peptidases Icp55 and Oct1 remove destabilizing amino-acid residues from the N termini of several preprotein intermediates according to the N-end rule of protein degradation [10] , [25] , [26] , [27] , [28] , [29] . The resulting double-processed proteins contain stabilizing N-terminal amino-acid residues and thus have a higher stability (longer half-life). The inner membrane protease (IMP) cleaves preproteins that carry bipartite presequences consisting of a positively charged N-terminal matrix-targeting signal and a hydrophobic inner membrane-sorting signal, which induces lateral release of the preprotein from the TIM23 complex into the lipid phase of the inner membrane. Bipartite presequences are first cleaved by MPP to remove the matrix-targeting signal, followed by removal of the sorting signal by IMP that carries its catalytic site on the intermembrane space side of the inner membrane [13] , [30] , [31] , [32] , [33] , [34] , [35] . These double-processed proteins are either released into the intermembrane space or are anchored in the inner membrane by a further hydrophobic segment located in the mature protein. For a few preproteins, N-terminal processing by proteases that are not specific for imported presequences has been observed, including the matrix-exposed m -AAA protease (Yta12-Afg3/Yta10) and the rhomboid protease Pcp1 that cleaves within the inner membrane [36] , [37] , [38] , [39] . We observed that the size of TIM23 SORT was altered in IMP yeast mutants, although none of the TIM23 subunits contains a bipartite presequence. Unexpectedly, Mgr2 carries a carboxy-terminal extension that functions as targeting sequence and is selectively cleaved by IMP, but not by other processing peptidases of mitochondria. Our work unveils processing of an unconventional C-terminal targeting signal as prerequisite for proper assembly and function of the mitochondrial presequence translocase. The TIM23 subunit Mgr2 is processed by IMP Upon lysis of mitochondria with the non-ionic detergent digitonin, blue native electrophoresis separates the TIM23 CORE complex from the slower migrating TIM23 SORT complexes ( Fig. 1a ) [14] , [17] , [20] . During analysis of TIM23 complexes in yeast-mutant mitochondria, we surprisingly noted that the gel mobility and abundance of the TIM23 SORT forms were altered in mitochondria lacking Imp1 ( Fig. 1a , lanes 2 and 4). TIM23 SORT of the mutant mitochondria migrated more slowly on the native gels and its levels were decreased, whereas the gel mobility and abundance of TIM23 CORE were not diminished (the levels of TIM23 CORE were even increased). Imp1 is one of the two catalytic subunits of IMP [26] , [30] , [31] , [32] , [34] . So far, none of the five subunits of the TIM23 complex has been known to be a substrate of IMP. Tim17 and Tim23 are synthesized as mature-sized proteins and are not proteolytically cleaved upon import into mitochondria [3] , [8] . Tim21 and Tim50 contain typical positively charged N-terminal presequences that are cleaved on the matrix side [10] , [14] , [40] , [41] , whereas Imp1 cleaves preproteins on the intermembrane space side of the inner membrane [13] , [30] , [32] , [33] , [34] , [35] . Tim21 and the recently identified Mgr2 are specifically present in the TIM23 SORT forms [14] , [17] , [20] . Mgr2 is proteolytically cleaved upon import into mitochondria [17] , however, neither processing site nor the responsible protease have been identified. We asked if processing of Mgr2 may be linked to Imp1 and thus may provide an explanation for the altered mobility of TIM23 SORT in imp1 Δ mitochondria. 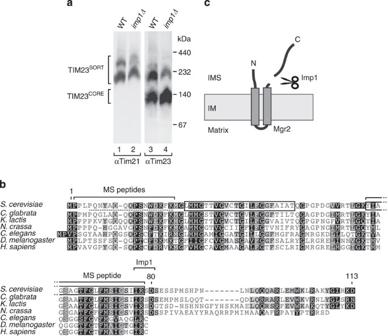Figure 1: Lack of Imp1 alters the gel mobility of native TIM23SORTcomplexes. (a) Blue native electrophoresis and western blot analysis of the presequence translocase (TIM23 complex) in mitochondria isolated from wild-type (WT) orimp1Δ yeast cells using antibodies against Tim21 and Tim23. The TIM23 core complex (TIM23CORE) and the Tim21-containing forms (TIM23SORT) are indicated. (b) Alignment of the yeast Mgr2 protein sequence (derived fromSaccharomycesGenome ORFYPL098C)17,47with Mgr2 orthologs from other fungi or metazoa (metazoan Mgr2 orthologs are also termed Romo1/MTGM)50,51. The background colours indicate similarity scores calculated according to the Blosum62 matrix: black, 100%; dark grey, 80–99%; light grey, 60–79%; white <60%. The dotted line indicates the peptide sequence used for generating antibodies against Mgr2. Continuous lines indicate the Mgr2 peptides identified by mass spectrometry (MS) of isolated TIM23 complexes. Boxes highlight the predicted transmembrane segments of Mgr2. The numbering of residues corresponds to the Mgr2 sequence fromS. cerevisiae. (c) Diagram of the predicted topology of Mgr2. IM, inner membrane; IMS, intermembrane space. Figure 1: Lack of Imp1 alters the gel mobility of native TIM23 SORT complexes. ( a ) Blue native electrophoresis and western blot analysis of the presequence translocase (TIM23 complex) in mitochondria isolated from wild-type (WT) or imp1 Δ yeast cells using antibodies against Tim21 and Tim23. The TIM23 core complex (TIM23 CORE ) and the Tim21-containing forms (TIM23 SORT ) are indicated. ( b ) Alignment of the yeast Mgr2 protein sequence (derived from Saccharomyces Genome ORF YPL098C ) [17] , [47] with Mgr2 orthologs from other fungi or metazoa (metazoan Mgr2 orthologs are also termed Romo1/MTGM) [50] , [51] . The background colours indicate similarity scores calculated according to the Blosum62 matrix: black, 100%; dark grey, 80–99%; light grey, 60–79%; white <60%. The dotted line indicates the peptide sequence used for generating antibodies against Mgr2. Continuous lines indicate the Mgr2 peptides identified by mass spectrometry (MS) of isolated TIM23 complexes. Boxes highlight the predicted transmembrane segments of Mgr2. The numbering of residues corresponds to the Mgr2 sequence from S. cerevisiae . ( c ) Diagram of the predicted topology of Mgr2. IM, inner membrane; IMS, intermembrane space. Full size image Mgr2 is a small inner membrane protein with two predicted transmembrane segments that are connected by a short loop ( Fig. 1b,c ) [17] . Mgr2 contains an N-terminal hydrophilic region of ~22 amino-acid residues (in front of the first predicted transmembrane segment) that may potentially function as cleavable presequence. However, mass spectrometric analysis of mature Mgr2 identified peptides that included residues 2–20 and 59–78 of the protein ( Fig. 1b ; Methods) and an antiserum raised against residues 5–20 of Mgr2 recognized the mature protein ( Fig. 2a ). These findings surprisingly indicated that the 12 kDa precursor of Mgr2 was not proteolytically processed at its N terminus (only the first methionine is removed) and thus had to be processed in its C-terminal region. The hydrophilic C-terminal region of Mgr2 located behind the second predicted transmembrane segment consists of ~35 residues. To date, C-terminal processing of a mitochondrial precursor protein has been reported only for the DNA helicase Hmi1, a matrix protein of 80 kDa loosely associated with the inner membrane [42] , [43] . It has been proposed that the last 14 C-terminal residues of Hmi1 are removed by MPP in the matrix [42] . To investigate if Mgr2 is a substrate of MPP, we made use of a mas1 yeast-mutant strain that contains a temperature-sensitive allele of the catalytic β-subunit of MPP [44] . Upon shift of the cells to non-permissive condition, mas1- mutant mitochondria accumulate the precursor forms of MPP-dependent mitochondrial proteins, shown here for the Rieske iron–sulphur protein by western blotting ( Fig. 2a ). In case of Mgr2, however, no accumulation of a precursor form was observed in mas1 -mutant mitochondria ( Fig. 2a ). 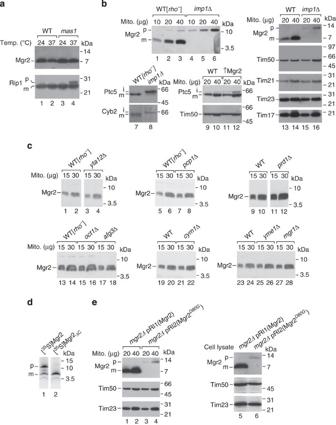Figure 2: Mgr2 is processed by the Imp1 protease. (a) Mitochondria were isolated from amas1temperature-sensitive mutant yeast strain and the corresponding wild type (WT) (either shifted to 37 °C for 6 h or further grown at 24 °C as indicated) and analysed by SDS–PAGE and western blotting with antibodies specific for Mgr2 or the Rieske iron–sulphur protein (Rip1). (b) Mitochondria from the BY4741rho−wild-type strain and theimp1Δ strain derived from the Euroscarf collection (lanes 1–8), the YPH499 strain transformed with the empty vector pRS426 and themgr2Δ strain transformed with pPGKMGR2(↑Mgr2) (lanes 9–12), and theimp1Δ strain GM103-4D31and the correspondingrho+wild-type (lanes 13–16) were subjected to SDS–PAGE and immunoblotting using the indicated antisera. Lanes 11 and 12, overexpression of Mgr2 led to a moderate accumulation of the intermediate form of Ptc5, whereas no precursor accumulation was observed for Tim50, which is processed on the matrix side40,41. (c) Mitochondria isolated from the indicated protease-deficient mutants and their corresponding wild-type strains were analysed as in (b). (d)35S-labelled Mgr2 and Mgr2ΔCprecursor proteins were incubated with isolated wild-type mitochondria. Samples were analysed by SDS–PAGE and digital autoradiography. (e) Centromeric plasmids encoding either wild-type Mgr2 (pRI1) or Mgr2D80G(pRI2) were used to transformmgr2Δ yeast cells. Isolated mitochondria (lanes 1–4) and total cell lysates (lanes 5 and 6) were analysed by SDS–PAGE and immunoblotting using antibodies specific for the indicated proteins. p, precursor; i, intermediate; m, mature. Figure 2: Mgr2 is processed by the Imp1 protease. ( a ) Mitochondria were isolated from a mas1 temperature-sensitive mutant yeast strain and the corresponding wild type (WT) (either shifted to 37 °C for 6 h or further grown at 24 °C as indicated) and analysed by SDS–PAGE and western blotting with antibodies specific for Mgr2 or the Rieske iron–sulphur protein (Rip1). ( b ) Mitochondria from the BY4741 rho − wild-type strain and the imp1 Δ strain derived from the Euroscarf collection (lanes 1–8), the YPH499 strain transformed with the empty vector pRS426 and the mgr2 Δ strain transformed with pPGK MGR2 (↑Mgr2) (lanes 9–12), and the imp1 Δ strain GM103-4D [31] and the corresponding rho + wild-type (lanes 13–16) were subjected to SDS–PAGE and immunoblotting using the indicated antisera. Lanes 11 and 12, overexpression of Mgr2 led to a moderate accumulation of the intermediate form of Ptc5, whereas no precursor accumulation was observed for Tim50, which is processed on the matrix side [40] , [41] . ( c ) Mitochondria isolated from the indicated protease-deficient mutants and their corresponding wild-type strains were analysed as in ( b ). ( d ) 35 S-labelled Mgr2 and Mgr2 Δ C precursor proteins were incubated with isolated wild-type mitochondria. Samples were analysed by SDS–PAGE and digital autoradiography. ( e ) Centromeric plasmids encoding either wild-type Mgr2 (pRI1) or Mgr2 D80G (pRI2) were used to transform mgr2 Δ yeast cells. Isolated mitochondria (lanes 1–4) and total cell lysates (lanes 5 and 6) were analysed by SDS–PAGE and immunoblotting using antibodies specific for the indicated proteins. p, precursor; i, intermediate; m, mature. Full size image We asked if Mgr2 was a substrate of the Imp1 protease. We used mitochondria isolated from imp1 Δ yeast strains. Processing of Mgr2 to the mature form was blocked and only the precursor form was observed in imp1 Δ mitochondria ( Fig. 2b , lanes 4–6, 15 and 16). The Imp1 substrates Ptc5 (mitochondrial phosphatase two C) and cytochrome b 2 accumulated as intermediate forms in imp1 Δ mutant mitochondria as reported ( Fig. 2b , lane 8) [30] , [31] , [32] , [34] , [35] . As lack of Imp1 causes a petite phenotype, that is, the mutant yeast cells are unable to grow on non-fermentable medium [32] , [34] , we used rho + as well as rho − wild-type mitochondria for comparison. Both wild-type mitochondria processed Mgr2 to the mature form independently of the petite phenotype ( Fig. 2b , lanes 1–3, 13 and 14). To exclude strain-specific differences, we compared imp1 Δ strains with different genotype backgrounds (see Methods) and observed the blocking of Mgr2 processing in each background ( Fig. 2b ). All other subunits of the TIM23 complex were processed to their mature forms in imp1 Δ mitochondria ( Fig. 2b , lanes 15 and 16), demonstrating that the role of Imp1 in biogenesis of the TIM23 complex was specific for Mgr2. We used a collection of yeast-mutant strains deficient in mitochondrial proteases that have been directly or indirectly implicated in the maturation of preproteins or protein quality control, including the mitochondrial intermediate peptidase Oct1, the rhomboid intramembrane protease Pcp1, the m -AAA protease (Yta12-Afg3/Yta10), the i -AAA protease (Yme1-Mgr1), and the oligopeptidases Prd1 and Cym1 (refs 11 , 24 , 36 , 37 , 38 , 39 , 45 , 46 , 47 ). In each case, Mgr2 was present in its mature form in mitochondria ( Fig. 2c ), indicating that none of the proteases was required for the processing of Mgr2. We conclude that the precursor of Mgr2 undergoes C-terminal processing by IMP without prior cleavage by MPP. As Mgr2 is specifically present in TIM23 SORT , the presence of the larger unprocessed Mgr2 in imp1 Δ mitochondria explains the mobility shift of TIM23 SORT on native gels. Imp1 processing site in the C-terminal region of Mgr2 Mutagenesis studies of Imp1 substrates revealed a consensus cleavage site that includes a hydrophobic non-aromatic residue at position −3 and an acidic residue at position +1 (refs 34 , 48 ). The residue requirement for position −1 is less stringent, as several structurally diverse residues allow cleavage [49] . We scanned the Mgr2 sequence for the presence of motifs that resemble the Imp1 consensus site. Saccharomyces cerevisiae Mgr2 contains four aspartates and two glutamates. Two of these residues, D80 and D113, are preceded by an isoleucine at position −3, fitting to an Imp1 consensus site. D113 is the last residue of yeast Mgr2 and removal of one residue is unlikely to account for the ~4 kDa apparent molecular mass difference between precursor and mature Mgr2 ( Fig. 2b ) [17] . Assuming that the processing site may be conserved, we aligned Mgr2 homologues of different species. The motif including D80, but not the motif including D113, was found to be conserved in fungal Mgr2 homologues ( Fig. 1b ). Remarkably, Mgr2 homologues in metazoa (also termed Romo1/MTGM) [50] , [51] not only lack the cleavage motif, but are C-terminally truncated compared with fungal Mgr2 homologues. D80 of yeast Mgr2 (and the corresponding residue in fungal homologues) represents the first residue of a C-terminal fungal extension that is absent in metazoa ( Fig. 1b ). These observations indicate that Imp1 may use the I77-D80 cleavage motif, that is, cleave yeast Mgr2 between residues 79 and 80. For an experimental assessment, we synthesized a truncated Mgr2 Δ C precursor lacking residues 80–113 and compared its SDS–PAGE mobility with wild-type Mgr2 that was processed in mitochondria. The gel mobility of both proteins was indistinguishable ( Fig. 2d ) in agreement with a cleavage after residue 79. To directly study the role of D80 in Mgr2 processing, we generated a yeast strain, in which wild-type Mgr2 was replaced by mutant Mgr2 harbouring a D80G substitution (a similar amino-acid replacement at the Imp1 site in the N-terminal part of cytochrome b 2 blocked cleavage) [48] . Mgr2 D80G was indeed not processed but accumulated in the precursor form ( Fig. 2e ). Taken together, we conclude that D80 is part of the Imp1 cleavage site of Mgr2 and that Imp1 removes the C-terminal extension of Mgr2 (residues 80–113), generating the mature-sized Mgr2 of 8 kDa. The second catalytic IMP subunit, Imp2, is active in imp1 Δ mitochondria [34] and its cleavage site specificity does not overlap with that of Imp1 (refs 32 , 34 , 48 ); as imp1 Δ mitochondria are blocked in Mgr2 processing, Imp2 does not process Mgr2. We will discuss below that the levels of unprocessed Mgr2 D80G were diminished in comparison with wild-type Mgr2 ( Fig. 2e ) like observed for unprocessed Mgr2 in imp1 Δ mitochondria ( Fig. 2b ) (the levels of other TIM23 subunits were not diminished). Mitochondrial levels of Mgr2 depend on C-terminal extension Does the C-terminal extension have a role in the biogenesis or function of Mgr2? We generated a yeast strain that expressed truncated Mgr2 Δ C lacking residues 80–113. Growth of the yeast-mutant strain was diminished on non-fermentable medium ( Fig. 3a ). The Mgr2 Δ C cells contained mature-sized Mgr2 comparably with cells expressing wild-type Mgr2 ( Fig. 3b ). However, the mitochondrial levels of Mgr2 were strongly reduced in Mgr2 Δ C cells, whereas the levels of other TIM23 subunits and further control proteins were not altered ( Fig. 3c ). Blue native electrophoresis revealed that the levels of TIM23 SORT complexes were strongly reduced in Mgr2 Δ C mitochondria; TIM23 CORE was not diminished ( Fig. 3d ). 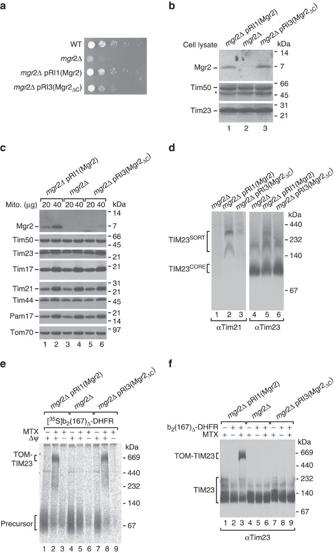Figure 3: The C-terminal cleavable extension is required for mitochondrial accumulation of Mgr2. (a) Serial dilutions of wild-type (WT) yeast cells transformed with the empty plasmid pRS414, andmgr2Δ cells transformed with either pRS414, the Mgr2-encoding plasmid pRI1, or the Mgr2ΔC-encoding plasmid pRI3 were spotted on glycerol-containing synthetic medium and grown at 24 °C. (b,c) Total cell lysates (b) or isolated mitochondria (c) obtained frommgr2Δ cells transformed with pRI1, pRS414, or pRI3 were analysed by SDS–PAGE and immunoblotting using the indicated antibodies. Asterisk, cross-reactive band. (d) Mitochondria described in panel (c) were lysed by 1% digitonin and subjected to blue native electrophoresis. TIM23COREand TIM23SORTcomplex forms were visualized with antibodies against Tim21 and Tim23. (e)35S-labelled b2(167)Δ-DHFR fusion protein was imported into mitochondria isolated frommgr2Δ cells transformed with either pRS414, pRI1, or pRI3 in the presence or absence of methotrexate (MTX). Where indicated the membrane potential (Δψ) of mitochondria was dissipated prior to the import reaction. Mitochondria were re-isolated, solubilized with digitonin buffer and analysed by blue native electrophoresis and digital autoradiography. TOM-TIM23, supercomplex of TOM and TIM23 translocases connected by the arrested precursor protein. (f) Isolated mitochondria from the indicated strains where incubated with or without 4 μg of recombinant, purified b2(167)Δ-DHFR fusion protein in the presence or absence of MTX. Subsequently, samples were processed as in (e), and Tim23-containing protein complexes were visualized by immunoblotting with a specific antiserum. Figure 3: The C-terminal cleavable extension is required for mitochondrial accumulation of Mgr2. ( a ) Serial dilutions of wild-type (WT) yeast cells transformed with the empty plasmid pRS414, and mgr2 Δ cells transformed with either pRS414, the Mgr2-encoding plasmid pRI1, or the Mgr2 Δ C -encoding plasmid pRI3 were spotted on glycerol-containing synthetic medium and grown at 24 °C. ( b , c ) Total cell lysates ( b ) or isolated mitochondria ( c ) obtained from mgr2 Δ cells transformed with pRI1, pRS414, or pRI3 were analysed by SDS–PAGE and immunoblotting using the indicated antibodies. Asterisk, cross-reactive band. ( d ) Mitochondria described in panel ( c ) were lysed by 1% digitonin and subjected to blue native electrophoresis. TIM23 CORE and TIM23 SORT complex forms were visualized with antibodies against Tim21 and Tim23. ( e ) 35 S-labelled b 2 (167)Δ-DHFR fusion protein was imported into mitochondria isolated from mgr2 Δ cells transformed with either pRS414, pRI1, or pRI3 in the presence or absence of methotrexate (MTX). Where indicated the membrane potential (Δψ) of mitochondria was dissipated prior to the import reaction. Mitochondria were re-isolated, solubilized with digitonin buffer and analysed by blue native electrophoresis and digital autoradiography. TOM-TIM23, supercomplex of TOM and TIM23 translocases connected by the arrested precursor protein. ( f ) Isolated mitochondria from the indicated strains where incubated with or without 4 μg of recombinant, purified b 2 (167)Δ-DHFR fusion protein in the presence or absence of MTX. Subsequently, samples were processed as in ( e ), and Tim23-containing protein complexes were visualized by immunoblotting with a specific antiserum. Full size image To analyse the function of Mgr2 in preprotein import into mitochondria, we studied the Mgr2-dependent formation of a TOM-TIM23-preprotein supercomplex in organello . This supercomplex is only formed when both translocases are properly assembled and functional, and thus can serve as sensitive assay for TIM23 assembly and activity [17] , [52] , [53] . A matrix-targeted fusion protein between an N-terminal portion of cytochrome b 2 and the passenger protein dihydrofolate reductase (b 2 (167) Δ -DHFR) [17] , [52] , [53] can be accumulated in mitochondrial import contact sites spanning TOM and TIM23 complexes. Unfolding of the C-terminal DHFR moiety is prevented by the ligand methotrexate, blocking complete translocation of the fusion protein into mitochondria; the cytochrome b 2 -portion is arrested in a TOM-TIM23 supercomplex that can be directly visualized by blue native electrophoresis ( Fig. 3e , lane 2; Fig. 3f , lane 3) [52] , [53] . Mgr2 is required for the stable preprotein-mediated connection of TOM and TIM23 complexes and thus in the absence of Mgr2 the supercomplex is not observed ( Fig. 3e , lane 5; Fig. 3f , lane 6) [17] . In Mgr2 Δ C mitochondria, we observed a differential result. When small radiochemical amounts of b 2 -DHFR were accumulated in mitochondrial import sites, formation of the TOM-TIM23-preprotein supercomplex was detected by autoradiography ( Fig. 3e , lane 8), demonstrating that Mgr2 lacking the C-terminal extension can function in preprotein import. However, when chemical amounts of the b 2 -DHFR fusion protein were used in order to saturate the mitochondrial import machinery, formation of the TOM-TIM23 supercomplex was not observed ( Fig. 3f , lane 9). In the latter assay, the TIM23 complex and its preprotein-dependent shift into the supercomplex were monitored by western blotting, whereas the radiochemical amounts of preprotein used in the first assay are so small that they cannot be detected by western blotting. We conclude that a small fraction of TIM23 complexes of Mgr2 Δ C mitochondria are assembled and functional, sufficient for the import of very small amounts of preproteins. The C-terminal extension is thus not strictly essential for assembly and proper function of Mgr2 in the TIM23 complex, but is critical for observing normal mitochondrial levels of Mgr2 and is therefore needed for mitochondrial preprotein import activity when larger amounts of preproteins are used. C-terminal extension of Mgr2 functions as targeting signal As Mgr2 Δ C cells expressed mature-sized Mgr2, yet the mitochondrial levels were strongly diminished ( Fig. 3b,c ), we asked if the C-terminal extension was required for the import of Mgr2 from the cytosol into mitochondria. We synthesized and radiolabelled the precursors of Mgr2 and truncated Mgr2 Δ C in yeast cytosolic extract ( Fig. 4a , lanes 1 and 2) and incubated them with isolated mitochondria. Wild-type [ 35 S]Mgr2 was imported into mitochondria and assembly into TIM23 SORT complexes was determined by blue native electrophoresis; the radiolabelled TIM23 SORT complexes were shifted in mitochondria containing protein A-tagged Tim23 or Tim21 ( Fig. 4a , lanes 3–8), demonstrating proper assembly of [ 35 S]Mgr2. Upon incubation of [ 35 S]Mgr2 Δ C with mitochondria, however, formation of radiolabelled TIM23 SORT complexes was inhibited ( Fig. 4a , lanes 9–12), supporting the view that the C-terminal extension was required for biogenesis of Mgr2. 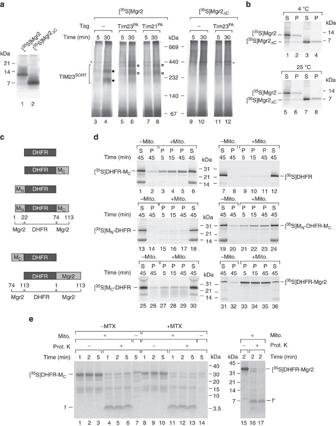Figure 4: The C-terminal extension of the Mgr2 precursor functions as mitochondrial-targeting signal. (a)35S-labelled Mgr2 or Mgr2ΔCprecursor proteins were analysed by SDS–PAGE (lanes 1 and 2). The precursors were imported intomgr2Δ mutant mitochondria harbouring protein A-tagged Tim23 or Tim21 as indicated. Samples were analysed by blue native electrophoresis and TIM23SORTcomplexes (closed and open circles) were detected by digital autoradiography (lanes 3–12). Asterisk, non-specific band. (b) The35S-labelled Mgr2 and Mgr2ΔCprecursor proteins were incubated for 15 min at 4 °C (lanes 1–4) or 25 °C (lanes 5–8). Aggregated (pellet, P) and soluble (supernatant, S) proteins were separated by centrifugation and detected by SDS–PAGE and autoradiography. Pellet, 100%; supernatant, 80%. (c) Schematic representation of the Mgr2–DHFR fusion proteins used in (d,e). MN, amino acids 1 to 22 of Mgr2 (N terminus); MC, amino acids 74 to 113 of the Mgr2 precursor (C terminus); Mgr2, full-length Mgr2 precursor (amino acids 1 to 113). (d) The different35S-labelled Mgr2–DHFR fusion proteins (or DHFR alone, lanes 7–12) were incubated in the presence or absence of wild-type mitochondria at 4 °C. After centrifugation at 20,000g, pellet (P) and supernatant (S) fractions were analysed by SDS–PAGE and autoradiography. Pellet, 100%; supernatant, 5%. (e)35S-labelled DHFR-MCwas incubated in the presence or absence of wild-type mitochondria at 25°C and subsequently treated with proteinase K (17 μg ml−1) as indicated (lanes 1-14).35S-labelled DHFR-Mgr2 was incubated with wild-type mitochondria at 25 °C (lanes 15–17). Where indicated, samples were treated with proteinase K (1.5–7.5 μg ml−1). All samples were analyzed by SDS–PAGE and autoradiography. f, f′, protease-protected fragments. Figure 4: The C-terminal extension of the Mgr2 precursor functions as mitochondrial-targeting signal. ( a ) 35 S-labelled Mgr2 or Mgr2 Δ C precursor proteins were analysed by SDS–PAGE (lanes 1 and 2). The precursors were imported into mgr2 Δ mutant mitochondria harbouring protein A-tagged Tim23 or Tim21 as indicated. Samples were analysed by blue native electrophoresis and TIM23 SORT complexes (closed and open circles) were detected by digital autoradiography (lanes 3–12). Asterisk, non-specific band. ( b ) The 35 S-labelled Mgr2 and Mgr2 Δ C precursor proteins were incubated for 15 min at 4 °C (lanes 1–4) or 25 °C (lanes 5–8). Aggregated (pellet, P) and soluble (supernatant, S) proteins were separated by centrifugation and detected by SDS–PAGE and autoradiography. Pellet, 100%; supernatant, 80%. ( c ) Schematic representation of the Mgr2–DHFR fusion proteins used in ( d , e ). M N , amino acids 1 to 22 of Mgr2 (N terminus); M C , amino acids 74 to 113 of the Mgr2 precursor (C terminus); Mgr2, full-length Mgr2 precursor (amino acids 1 to 113). ( d ) The different 35 S-labelled Mgr2–DHFR fusion proteins (or DHFR alone, lanes 7–12) were incubated in the presence or absence of wild-type mitochondria at 4 °C. After centrifugation at 20,000 g , pellet (P) and supernatant (S) fractions were analysed by SDS–PAGE and autoradiography. Pellet, 100%; supernatant, 5%. ( e ) 35 S-labelled DHFR-M C was incubated in the presence or absence of wild-type mitochondria at 25°C and subsequently treated with proteinase K (17 μg ml −1 ) as indicated (lanes 1-14). 35 S-labelled DHFR-Mgr2 was incubated with wild-type mitochondria at 25 °C (lanes 15–17). Where indicated, samples were treated with proteinase K (1.5–7.5 μg ml −1 ). All samples were analyzed by SDS–PAGE and autoradiography. f, f′, protease-protected fragments. Full size image As mature Mgr2 is a small hydrophobic protein, we wondered if the hydrophilic C-terminal extension was involved in maintaining the cytosolic precursor in a soluble form and thus prevented its aggregation. We synthesized Mgr2 and Mgr2 ΔC precursors in yeast cytosolic extracts, incubated them at different temperatures and separated soluble and aggregated proteins by centrifugation. Both Mgr2 and Mgr2 Δ C showed a similar, low propensity for aggregation ( Fig. 4b ), indicating that the C-terminal extension does not have a critical role in keeping the cytosolic precursor in a soluble state. We asked if the C-terminal extension of Mgr2 functions as targeting signal. Mitochondrial-targeting signals are typically positively charged [3] , [4] , [8] , [9] , [10] , [11] . The C-terminal extensions of fungal Mgr2 proteins contain positively and negatively charged amino-acid residues, but show an overall net positive charge ( Fig. 1b ). We fused the C-terminal extension to the C terminus of the passenger protein DHFR. The resulting fusion protein DHFR-M C ( Fig. 4c ) bound to mitochondria in a time-dependent manner in contrast to DHFR alone ( Fig. 4d , upper panels). The (non-cleavable) N-terminal hydrophilic region of Mgr2 also contains positively and negatively charged residues with an overall net positive charge ( Fig. 1b ) and may thus also function as a targeting signal. We constructed a fusion protein carrying the N-terminal 22 residues of Mgr2 in front of DHFR ( Fig. 4c ). However, M N -DHFR did not show any appreciable binding to mitochondria ( Fig. 4d , lanes 15–17) and the double fusion protein M N -DHFR-M C bound to mitochondria in a manner comparable with the single DHFR-M C fusion protein ( Fig. 4d , lanes 21–23). The fusion protein M C -DHFR, which carries the C-terminal extension of Mgr2 at the N terminus of DHFR, bound to mitochondria only marginally ( Fig. 4c , d , lower left panel), indicating that the extension of Mgr2 functions as C-terminal targeting sequence. When mitochondria with bound [ 35 S]DHFR-M C were treated with protease, a fragment of ~4 kDa was generated ( Fig. 4e , lanes 4–6). The fragment was not generated in the absence of mitochondria ( Fig. 4e , lane 7). The size of the fragment corresponds to the size of the C-terminal extension of Mgr2. To exclude that the fragment was derived from DHFR, we stabilized the folding of the DHFR moiety by methotrexate [8] , [52] , [53] . The protease-protected fragment was generated independently of the presence or absence of methotrexate ( Fig. 4e , compare lanes 11–13 with lanes 4–6), strongly supporting the view that the fragment was derived from the Mgr2 portion of DHFR-M C , not from DHFR. For comparison, we generated a fusion protein consisting of DHFR and the full-length Mgr2 precursor that efficiently bound to mitochondria ( Fig. 4c , lower right panel). Protease treatment of mitochondria generated a protected fragment of ~8 kDa, similar to the size of mature Mgr2 ( Fig. 4e , lanes 16 and 17). These results indicate that the full-length Mgr2 precursor and the C-terminal extension target attached DHFR to mitochondria, but do not direct the DHFR moiety to a protease-protected location inside mitochondria; only the Mgr2 portion is transported into mitochondria. The Mgr2 import pathway thus differs from the classical presequence import pathway into mitochondria, where the import-driving activity of the matrix-exposed import motor [3] , [4] , [21] promotes the unfolding of DHFR (in the absence of methotrexate), leading to the complete translocation of DHFR fusion proteins into mitochondria [52] , [53] . Taken together, the C-terminal extension, but not the N-terminal region of Mgr2 efficiently targets DHFR to mitochondria, demonstrating that the C-terminal extension functions as mitochondrial-targeting sequence. C-terminal processing of Mgr2 promotes TIM23 assembly Figure 2b,e showed that Mgr2 was unprocessed in imp1 Δ and Mgr2 D80G mitochondria and that its levels were strongly reduced in both mutant mitochondria. Consequently, the steady-state levels of TIM23 SORT were reduced when Mgr2 could not be processed (Mgr2 D80G mitochondria; Fig. 5a ). Upon incubation of the non-cleavable 35 S-labelled Mgr2 D80G precursor with mitochondria, formation of radiolabelled TIM23 SORT complexes was impaired, but not blocked. The amounts of radiolabelled TIM23 SORT were diminished and the blue native migration pattern was shifted ( Fig. 5b , lane 2 and quantification). A comparable shift of TIM23 SORT and diminished assembly efficiency were observed when the wild-type Mgr2 precursor or Mgr2 D80G were imported into imp1 Δ mitochondria ( Fig. 5b , lanes 3 and 4). We conclude that unprocessed Mgr2 assembles into TIM23 SORT with lower efficiency. 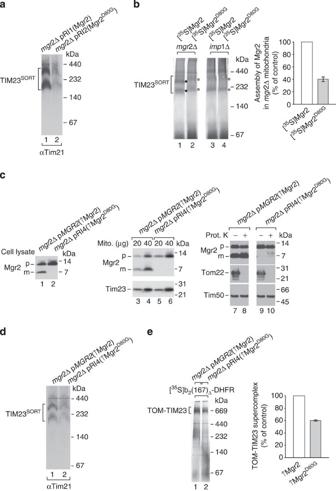Figure 5: Removal of the Mgr2 C-terminal targeting signal is required for TIM23 complex assembly and function. (a) Mitochondria isolated frommgr2Δ cells transformed with plasmids pRI1 (Mgr2) or pRI2 (Mgr2D80G) were lysed with digitonin and analysed by blue native electrophoresis and immunoblotting using an antibody against Tim21 to detect TIM23SORTcomplexes. (b) Radiolabelled Mgr2 or Mgr2D80Gprecursor proteins were imported intomgr2Δ (lanes 1 and 2) orimp1Δ (lanes 3 and 4) mutant mitochondria. Upon lysis with digitonin and blue native electrophoresis, TIM23SORTcomplexes were visualized by digital autoradiography (closed and open circles). The assembly of Mgr2 and Mgr2D80Ginmgr2Δ mitochondria was quantified. Assembled Mgr2 was set to 100% (control). Data values of Mgr2D80Gare shown as mean±s.e.m. (n=3). (c) Total cell lysates (lanes 1 and 2) or isolated mitochondria (lanes 3–10) obtained frommgr2Δ cells transformed with the high copy number plasmids pPGKMGR2(pMGR2↑Mgr2) or pRI4 (↑Mgr2D80G) were analysed by SDS–PAGE and immunoblotting using the indicated antisera. Where indicated, mitochondria were treated with 5 μg ml−1proteinase K. p, precursor; m, mature. (d) Isolated digitonin-solubilized mitochondria as indicated were subjected to blue native electrophoresis and immunoblotting with anti-Tim21 antiserum. (e)35S-labelled b2(167)Δ-DHFR fusion protein was imported into the indicated mitochondria in the presence of methotrexate, leading to the formation of TOM-TIM23-precursor supercomplexes. Samples were processed and analysed as in (b). The amount of supercomplex formed in ↑Mgr2 mitochondria was set to 100% (control). Data values of ↑Mgr2D80Gmitochondria are shown as mean±s.e.m. (n=4). Figure 5: Removal of the Mgr2 C-terminal targeting signal is required for TIM23 complex assembly and function. ( a ) Mitochondria isolated from mgr2 Δ cells transformed with plasmids pRI1 (Mgr2) or pRI2 (Mgr2 D80G ) were lysed with digitonin and analysed by blue native electrophoresis and immunoblotting using an antibody against Tim21 to detect TIM23 SORT complexes. ( b ) Radiolabelled Mgr2 or Mgr2 D80G precursor proteins were imported into mgr2 Δ (lanes 1 and 2) or imp1 Δ (lanes 3 and 4) mutant mitochondria. Upon lysis with digitonin and blue native electrophoresis, TIM23 SORT complexes were visualized by digital autoradiography (closed and open circles). The assembly of Mgr2 and Mgr2 D80G in mgr2 Δ mitochondria was quantified. Assembled Mgr2 was set to 100% (control). Data values of Mgr2 D80G are shown as mean±s.e.m. ( n =3). ( c ) Total cell lysates (lanes 1 and 2) or isolated mitochondria (lanes 3–10) obtained from mgr2 Δ cells transformed with the high copy number plasmids pPGK MGR2 (p MGR2 ↑Mgr2) or pRI4 (↑Mgr2 D80G ) were analysed by SDS–PAGE and immunoblotting using the indicated antisera. Where indicated, mitochondria were treated with 5 μg ml −1 proteinase K. p, precursor; m, mature. ( d ) Isolated digitonin-solubilized mitochondria as indicated were subjected to blue native electrophoresis and immunoblotting with anti-Tim21 antiserum. ( e ) 35 S-labelled b 2 (167)Δ-DHFR fusion protein was imported into the indicated mitochondria in the presence of methotrexate, leading to the formation of TOM-TIM23-precursor supercomplexes. Samples were processed and analysed as in ( b ). The amount of supercomplex formed in ↑Mgr2 mitochondria was set to 100% (control). Data values of ↑Mgr2 D80G mitochondria are shown as mean±s.e.m. ( n =4). Full size image Two possibilities were conceivable for the underlying molecular mechanism: either unprocessed Mgr2 was rapidly degraded upon import in mitochondria and therefore not available in sufficient amounts for assembly into TIM23 SORT ; or, the presence of the C-terminal Mgr2 extension impaired stable assembly of TIM23 SORT and thus not properly assembled, unprocessed Mgr2 was eventually degraded. To distinguish between these possibilities, we generated yeast strains that expressed Mgr2 D80G as well as wild-type Mgr2 from high copy number plasmids such that the cellular and mitochondrial levels of Mgr2 D80G and Mgr2 were comparable ( Fig. 5c ). The amount of Tim23 SORT detected in the strain overexpressing Mgr2 D80G was diminished ( Fig. 5d ), providing evidence for the second mechanism that is, stable assembly of unprocessed Mgr2 D80G was inhibited despite the presence of sufficient amounts of the protein in mitochondria. To test the function of Tim23 SORT complexes containing Mgr2 D80G , we accumulated small radiochemical amounts of b 2 (167)Δ-DHFR in TOM-TIM23 supercomplexes and observed a significant reduction of supercomplex formation in the mutant mitochondria ( Fig. 5e ). This result is in contrast to the observation with Mgr2 Δ C mitochondria where the reduced amounts of TIM23 SORT complexes did not impair the formation of TOM-TIM23 supercomplexes with radiochemical amounts of preprotein ( Fig. 3e ). Taken together, the presence of the C-terminal extension of Mgr2 inhibits proper assembly and function of TIM23 SORT and thus impairs the activity of the presequence translocase in preprotein import. We report a new mechanism for biogenesis and assembly of the mitochondrial presequence translocase. Mgr2, a subunit of the TIM23 SORT complex, is targeted to mitochondria by a cleavable C-terminal extension ( Fig. 1c ). Upon import, the targeting sequence has to be proteolytically removed by the inner membrane-located Imp1 protease as prerequisite for proper assembly and function of the translocase. Thus, lack of the C-terminal targeting sequence as well as defective proteolytic removal of the sequence reduce the mitochondrial levels of Mgr2. IMP has been known to proteolytically process a number of nuclear-encoded mitochondrial proteins as well as the mitochondrial-encoded Cox2 protein, however, in each case, IMP cleaved an N-terminal presequence [11] , [13] , [24] , [31] . We report the first identification of a C-terminal mitochondrial-targeting signal that is exclusively processed by IMP. Mgr2 contains hydrophilic regions with a net positive charge at both termini, however, only the C-terminal extension is able to target a passenger protein to mitochondria. The C-terminal targeting sequence is found in the fungal homologues of Mgr2, but not in metazoa, suggesting that the C-terminal signal promotes efficient targeting of Mgr2 in rapidly growing cells, but is not required in more slowly growing cells. In support of this view, deletion of the C-terminal signal strongly reduced the mitochondrial levels of Mgr2, but did not fully block translocation of Mgr2 into mitochondria. Thus, the mature part of Mgr2 contains targeting information of low efficiency also in yeast. Mgr2 lacking the C-terminal signal was imported into mitochondria with low yield ( Fig. 3c ), yet the small amounts of imported Mgr2 were correctly assembled and functional in the presequence translocase, indicating that the C-terminal extension is required for efficient targeting to mitochondria but not for assembly and activity of Mgr2 in the TIM23 complex. Although N-terminal processing of mitochondrial presequences has been widely studied [3] , [4] , [10] , [11] , [12] , [23] , [25] , [36] , [37] , [38] , [39] , [54] , C-terminal processing of mitochondrial-targeting signals is a largely unexplored field. So far, one case of processing of a C-terminal mitochondrial-targeting sequence has been reported [42] , [43] . The C-terminal ~36 residues of Hmi1 can function as targeting signal. Upon import into the matrix, only part of the targeting sequence, ~14 C-terminal residues, are presumably removed by MPP [42] . The function of C-terminal processing of Hmi1 is unknown. We found that in case of Mgr2 the entire C-terminal-targeting sequence is proteolytically removed. The reason is that the Mgr2-targeting sequence interferes with assembly and activity of the TIM23 SORT complex. A permanent presence of the C-terminal extension in a cleavage-defective mutant impairs stable assembly and function of the presequence translocase and disturbs the cooperation of TOM and TIM23 complexes in preprotein import. C-terminal processing of Mgr2 by IMP is thus crucial for proper assembly of the TIM23 complex. Taken together, we report an unanticipated role of IMP for biogenesis and function of the mitochondrial presequence translocase. IMP mediates processing of an unconventional C-terminal targeting sequence and thus promotes stable assembly and function of this main translocase of the inner mitochondrial membrane. Yeast strains and growth conditions The following S. cerevisiae strains were used: YPH499 ( MATa , ade2-101 , his3-Δ200 , leu2-Δ1 , ura3-52 , trp1-Δ63, lys2-801 ), JRY675WT ( MATa , ura3-52 , leu2Δ , his4-519 ), BY4741 ( MATa , his3Δ1 , leu2Δ0 , met15Δ0, ura3Δ0 ), BY4741 rho − (ref. 55 ) and a mas1 temperature-sensitive mutant ( Matα , ura3-52 , trp1-1 , leu2-3 , leu2-112 , his3-11 , his3-15 ) together with the corresponding wild type [44] . The mgr2Δ deletion mutant as well as strains containing a deletion of MGR2 and expressing either protein A-tagged Tim23 or protein A-tagged Tim21 were described [17] . The imp1Δ deletion mutant GM103-4D has been described by Behrens et al. [31] . A second imp1Δ as well as the deletion strains yta12Δ , pcp1Δ , prd1Δ , oct1Δ , afg3Δ , cym1Δ , yme1Δ and mgr1Δ were obtained from Euroscarf (corresponding open reading frames replaced by a kanamycin resistance cassette in the wild-type strain BY4741). Strains imp1Δ , yta12Δ , pcp1Δ , prd1Δ , oct1Δ , afg3Δ , cym1Δ , yme1Δ and the corresponding wild-type strains were grown at 24 °C on fermentable (1% (w/v) yeast extract, 2% (w/v) bacto peptone, 2% (w/v) sucrose, pH 5.0) or non-fermentable (3% (w/v) glycerol instead of sucrose) medium. The mas1 -mutant and wild-type cells were shifted to the non-permissive temperature of 37 °C for 6 h prior to isolation of mitochondria. Re-expression of wild-type Mgr2 or expression of Mgr2-mutant variants was achieved by transforming mgr2 Δ yeast cells with plasmids pPGK MGR2 (ref. 17 ), pRI1, pRI2, pRI3 or pRI4 (see below). Control strains expressing wild-type Mgr2 from its chromosomal locus were obtained by transforming YPH499 with the empty vectors pRS414 or pRS426. Control strains lacking Mgr2 were obtained by transforming mgr2 Δ cells with pRS414. For isolation of mitochondria, cells were grown at 30 °C in synthetic defined medium containing 0.67% Bacto-yeast nitrogen base, dropout amino-acid mix, 3% glycerol and 0.2% glucose. Plasmids The plasmid pPGK MGR2 has been described [17] . For generation of plasmid pRI1, a DNA fragment corresponding to nucleotides −306 to +647 with respect to the MGR2 start codon, including the MGR2 promoter, open reading frame and terminator, was amplified by polymerase chain reaction (PCR) and cloned into pRS414 using the Eco RI restriction site. The Mgr2D80G mutation was introduced by QuikChange mutagenesis (Stratagene) into pRI1 yielding pRI2 and into pPGK MGR2 generating pRI4. A deletion of the MGR2 codons 80–113 was introduced into pRI1 by QuikChange mutagenesis to generate pRI3 for expression of Mgr2 Δ C . Plasmid pUHE73-1 encoding a b 2 (167)Δ-DHFR fusion protein, which consists of the N-terminal part of cytochrome b 2 (lacking the hydrophobic inner membrane-sorting signal, amino-acid residues 47 to 65) and the passenger protein DHFR, has been described [52] . Constructs encoding Mgr2–DHFR fusion proteins were generated as follows. The mouse DHFR open reading frame (ORF) was cloned downstream of the SP6 promoter sequence into a pGEM-4Z vector (Promega) using the BamHI restriction site, generating pDHFR. A construct encoding M N -DHFR was generated by PCR from pDHFR using a DHFR ORF upstream oligonucleotide, which contains a 5′ non-annealing region corresponding to the sequence encoding the Mgr2 amino-acid residues 1 to 22, and a DHFR ORF downstream oligonucleotide. This fragment was cloned into pGEM-4Z using the Eco RI and Xba I restriction sites to generate plasmid pM N -DHFR. A DNA fragment encoding the Mgr2 amino-acid residues 74 to 113 was amplified by PCR from YPH499 genomic DNA and fused by overlap extension PCR (either upstream or downstream) to a DNA fragment encoding DHFR only. The resulting PCR products were digested with Eco RI and Xba I and cloned into pGEM-4Z yielding plasmids pM C -DHFR and pDHFR-M C , respectively. DNA fragments encoding the full-length Mgr2 precursor or the Mgr2 amino-acid residues 74 to 113 were fused by overlap extension PCR (downstream) to a DNA fragment encoding DHFR only or DHFR C-terminally fused to Mgr2 residues 1 to 22, respectively. The resulting PCR products were digested with Eco RI and Xba I and cloned into pGEM-4Z yielding plasmids pDHFR-Mgr2 and pM N -DHFR-M C . Protein import into mitochondria Isolated mitochondria were obtained by differential centrifugation [56] . For the in vitro synthesis of radiolabelled Mgr2 or Mgr2 D80G precursor proteins, the corresponding DNA sequences were amplified from plasmids pRI1 and pRI2, respectively, fused to the SP6 promoter sequence and transcribed using the mMESSAGE mMACHINE SP6 kit (Invitrogen). mRNA was purified with the MEGAclear kit (Invitrogen) and translated in a yeast cytosolic extract [57] in the presence of [ 35 S]methionine. Radiolabelled DHFR and different Mgr2–DHFR fusion proteins were synthesized using a transcription/translation reticulocyte lysate system (GE Healthcare) and plasmids pDHFR, pM N -DHFR, pDHFR-M C , pM N -DHFR-M C , pM C -DHFR and pDHFR-Mgr2. Chemical amounts of the b 2 (167)Δ-DHFR precursor were produced by recombinant expression in Escherichia coli and purification via ion exchange chromatography [52] . For in vitro import experiments, precursor proteins were added to mitochondria in import buffer (3% (w/v) fatty acid-free BSA, 250 mM sucrose, 80 mM KCl, 5 mM MgCl 2 , 2 mM KH 2 PO 4 , 5 mM methionine and 10 mM MOPS-KOH, pH 7.2) in the presence of 2 mM NADH, 2 mM ATP and an ATP- regenerating system (5 mM creatine phosphate and 0.1 mg ml −1 creatine kinase). Where indicated 5 μM methotrexate was added. Import reactions were stopped by adding AVO mix (8 μM antimycin A, 1 μM valinomycin and 20 μM oligomycin, final concentrations) and cooling on ice. Mitochondria were washed with SEM buffer (1 mM EDTA, 250 mM sucrose, 10 mM MOPS-KOH, pH 7.2) and analysed by SDS–PAGE or blue native electrophoresis. Radioactive protein bands were detected by digital autoradiography. Non-relevant lanes were removed by digital processing (indicated by white separating line). Quantification of radioactive signals and image processing were performed using the Multi Gauge software (Fujifilm). Full scans of gel autoradiographs and western blots are shown in Supplementary Fig. S1 . Total cell and mitochondrial protein analysis To prepare total cell extracts, 10 mg of yeast cells (wet weight) were harvested, resuspended in 1 ml 250 mM NaOH supplemented with 0.15 mM 2-mercaptoethanol, incubated on ice for 10 min, and subjected to TCA precipitation. Mitochondrial proteins or protein complexes were separated by SDS–PAGE or blue native electrophoresis. Where indicated, samples were treated with proteinase K at 4 °C, followed by addition of phenylmethylsulfonyl fluoride. For SDS–PAGE, samples were resuspended in lysis buffer (2% (w/v) SDS, 10% (v/v) glycerol, 60 mM Tris-HCl, pH 6.8, 0.01% (w/v) bromophenol blue, 2 mM PMSF). For blue native electrophoresis, mitochondria were washed with SEM buffer and solubilized in ice-cold solubilization buffer (1% (w/v) digitonin, 20 mM Tris-HCl, pH 7.4, 0.1 mM EDTA, 50 mM NaCl, and 10% (v/v) glycerol) for 15 min on ice [52] , [58] . Samples were subjected to a clarifying centrifugation, the supernatants were mixed with ice-cold blue native loading buffer (5% (w/v) Coomassie brilliant blue G-250, 100 mM Bis-Tris-HCl, pH 7.0 and 500 mM 6-aminocaproic acid) and loaded onto 6–16.5% polyacrylamid gradient blue native gels. Protein aggregation assay Aggregation propensities of in vitro synthesized proteins were assessed according to Goloubinoff et al. [59] In brief, radiolabelled Mgr2 or Mgr2 Δ C were synthesized in yeast cytosolic extract, and translation reactions were subjected to a clarifying spin for 15 min at 20,000 g . The supernatant was subsequently diluted fourfold in aggregation buffer (50 mM Hepes-KOH, pH 7.6, 150 mM KCl, 20 mM MgCl 2 , 10 mM DTT, 10 mM ATP) and incubated at 4 °C or 25 °C for 15 min. Samples were then centrifuged for 15 min at 20,000 g to separate aggregated proteins (pellet fraction) from soluble proteins (supernatant fraction). Mass spectrometry and sequence analysis TIM23 complexes were isolated by immunoglobulin G affinity chromatography [17] via protein A-tagged Tim21. Proteolytic digestion and mass spectrometric analysis of purified TIM23 complexes [17] yielded the tryptic Mgr2 peptides PPLPQNYAQQQPSNWDK (residues 2–18), PPLPQNYAQQQPSNWDKFK (residues 2–20) and YIAGSAGTFGLFMSIGSIIR (residues 59–78) (each one identified in four independent experiments; false discovery rate <1%). Mgr2/Romo1 amino-acid sequence alignments were generated using Geneious 5.4.3 software and the Blosum62 score matrix. Values of amino-acid residue similarities in Mgr2 ortholog sequences were calculated according to the Blosum62 score matrix. Yeast Mgr2 transmembrane segments were predicted using the Hydropathy-Plot MPEx software [60] . How to cite this article: Ieva, R. et al. Mitochondrial inner membrane protease promotes assembly of presequence translocase by removing a carboxy-terminal targeting sequence. Nat. Commun. 4:2853 doi: 10.1038/ncomms3853 (2013).